Efficient and selective photocatalytic CH4conversion to CH3OH with O2by controlling overoxidation on TiO2 The conversion of photocatalytic methane into methanol in high yield with selectivity remains a huge challenge due to unavoidable overoxidation. Here, the photocatalytic oxidation of CH 4 into CH 3 OH by O 2 is carried out on Ag-decorated facet-dominated TiO 2 . The {001}-dominated TiO 2 shows a durable CH 3 OH yield of 4.8 mmol g −1 h −1 and a selectivity of approximately 80%, which represent much higher values than those reported in recent studies and are better than those obtained for {101}-dominated TiO 2 . Operando Fourier transform infrared spectroscopy, electron spin resonance, and nuclear magnetic resonance techniques are used to comprehensively clarify the underlying mechanism. The straightforward generation of oxygen vacancies on {001} by photoinduced holes plays a key role in avoiding the formation of •CH 3 and •OH, which are the main factors leading to overoxidation and are generally formed on the {101} facet. The generation of oxygen vacancies on {001} results in distinct intermediates and reaction pathways (oxygen vacancy → Ti–O 2 • → Ti–OO–Ti and Ti–(OO) → Ti–O • pairs), thus achieving high selectivity and yield for CH 4 photooxidation into CH 3 OH. Direct conversion of CH 4 into methanol (CH 3 OH) is one of the most promising methods for methane optimization and utilization. However, CH 4 is a very stable and inert molecule due to its negligible electron affinity, low polarizability, and high bonding energy for C–H (the first dissociation energy at 439 kJ mol −1 ). Thus, high temperatures and pressures are normally required to activate C–H bonds, which greatly increases capital investment and gives rise to operational risks and environmental problems [1] . Photocatalysis is a potential way to drive CH 4 oxidation by utilizing photon energy instead of thermal energy. Upon excitation of semiconducting photocatalysts by photons, a series of highly active oxygen-containing radicals formed in photocatalytic CH 4 oxidation can readily activate the C–H bond at room temperature [2] , [3] , [4] , [5] , [6] . However, the activation energy of the C–H bond in CH 4 is much higher than that in the product (CH 3 OH) [7] . Thus, after the first C–H bond of CH 4 is activated by active free radicals to form methyl or methoxy species, these species are easier to be activated and oxidized than CH 4 , eventually resulting in overoxidation of CH 3 OH to produce CO and CO 2 [8] . Especially for gas-phase CH 4 oxidation, the product CH 3 OH can easily adsorb onto the surface of photocatalyst (such as TiO 2 and ZnO loaded with various cocatalysts) and become overoxidized to CO and CO 2 [9] , [10] , [11] . Due to unavoidable overoxidation, achieving high activity along with high selectivity at the same time is barely realized in the photocatalytic oxidation of CH 4 to CH 3 OH [12] , [13] , [14] . The enhancement of one usually sacrifices the other. It has been found that in aqueous-phase CH 4 oxidation, water can promote the desorption of products from active sites to avoid serious overoxidation [15] , [16] . Recently, Ma and Tang et al. [17] reported direct photocatalysis of CH 4 into CH 3 OH using a FeO x /TiO 2 catalyst with H 2 O 2 as the oxidant in an aqueous-phase system, resulting in a high CH 3 OH selectivity of ~90% but a relatively low yield of ~352 µmol g −1 h −1 . However, the relatively high cost of H 2 O 2 greatly limits its commercial application. Using O 2 instead of H 2 O 2 as the economically viable oxidant would represent substantial progress towards the oxidation of CH 4 [1] . In this case, Ye and coworkers [2] used molecular O 2 to photooxidize CH 4 on Au/ZnO with a total organic compound selectivity of 95%. However, the CH 3 OH product tends to be overoxidized by •OH radicals formed in the reaction, which results in a CH 3 OH selectivity of less than 27% with a yield of 2.0 mmol g −1 h −1 . More recently, Ye and coworkers used a CrO x -decorated Au/TiO 2 photocatalyst to reduce the formation of •OH radicals in the reaction [18] , which increased the selectivity of CH 3 OH to ~50% with a yield of 2.5 mmol g −1 h −1 . As such, the overoxidation of CH 3 OH should be partly attributed to the formation of •OH radicals. Furthermore, for the reported catalysts, CH 4 can react with the photoinduced holes to form •CH 3 on the surface, and the •CH 3 can react with O 2 and superoxide (O 2 • − ) to mainly form CH 3 OOH rather than CH 3 OH [2] , [6] , [19] . It should be noted that CH 3 OOH can readily decompose into HCHO and H 2 O [2] , [9] . Therefore, as long as •CH 3 and •OH exist in photocatalytic CH 4 oxidation, it is difficult to improve the selectivity of CH 3 OH unless a new reaction pathway is introduced to reduce the formation of •CH 3 and •OH through rational catalyst design. It has been reported that the intermediate photocatalytic species are closely related to the arrangement and coordination of the surface atoms on different crystal facets [20] , [21] , [22] , [23] , [24] . In this work, two types of anatase TiO 2 , {001} or {101}-dominated TiO 2 with Ag cocatalysts, are studied for CH 4 photooxidation by O 2 . The {001}-dominated TiO 2 shows a durable CH 3 OH yield of 4.8 mmol/g/h and a selectivity of ~80%, which are much higher values than those obtained on {101}-dominated TiO 2 . A comprehensive study by operando IR, ESR, and NMR reveals that the initial generation of oxygen vacancies on {001} by photoinduced holes can avoid the formation of •CH 3 and •OH in the following reaction steps (Ti–O 2 • → Ti–OO–Ti and Ti–(OO) → Ti–O • pairs) to significantly reduce overoxidation. The scarcity of photogenerated oxygen vacancies on {101} leads to the formation of •CH 3 and •OH, which is the main factor for overoxidation. This study provides a strategy to avoid overoxidation in reforming CH 4 to CH 3 OH using other photocatalysts by controlling the generation of photogenerated oxygen vacancies. Selective photocatalytic oxidation of CH 4 to CH 3 OH Two types of anatase TiO 2 (Supplementary Fig. S1 ) with predominantly exposed {001} or {101} facets were prepared, called TiO 2 {001} and TiO 2 {101} , respectively. Silver (Ag) was chosen to decorate TiO 2 , which can trap photoinduced electrons to facilitate the separation and transfer of photoinduced carriers [25] , [26] , [27] . Typical oxide semiconductors, such as ZnO and TiO 2 , loaded with Ag cocatalysts have been demonstrated to exhibit good photocatalytic activity for CH 4 activation [10] , [28] . Bare TiO 2 (including TiO 2 {001} and TiO 2 {101} ) and that with variable Ag loading were evaluated for photocatalytic CH 4 oxidation with molecular O 2 as an oxidant (CH 4 :O 2 ratio = 20:1). As shown in Fig. 1A , the products of CH 4 photooxidation on TiO 2 {001} are CH 3 OH, HCHO, CO, and CO 2 . Among these products, the yield of CH 3 OH is 950 µmol g cat. −1 h −1 and the selectivity of CH 3 OH is 42%. However, only deep oxidation products (HCHO, CO, and CO 2 ) are formed on TiO 2 {101} , and the production of CH 3 OH is invisible (Fig. 1B ). This is consistent with previous reports of CH 4 photooxidation by O 2 over TiO 2 (P25) and ZnO [2] , [9] . As such, the {001} facet should be favorable for the formation of CH 3 OH in CH 4 photooxidation by O 2 , while the {101} facet is inclined to undergo deep oxidation. Fig. 1: Photocatalytic CH 4 conversion with molecular O 2 . CH 3 OH selectivity and product yields for a series of Ag-loaded TiO 2 photocatalysts with predominantly exposed A {001} facets (0–5.0%Ag/TiO 2 {001} ) and B {101} facets (0–3.0%Ag/TiO 2 {101} ) under 2 h of irradiation. Time course for CH 3 OH selectivity and product yields for C 3.2%Ag/TiO 2 {001} and D 2.1%Ag/TiO 2 {101} under irradiation. Reaction conditions: 10 mg Ag/TiO 2 , 100 mL water, 2 MPa CH 4 , 0.1 MPa O 2 , 25 °C, light source: 300 W Xe lamp, light intensity of 450 mW/cm 2 . Full size image We further studied the effect of the Ag loading amount on the catalytic performance. Clearly, a series of Ag loadings on TiO 2 can effectively improve the activity of CH 4 photooxidation. For TiO 2 {001} , a 2.5%Ag and 3.2%Ag loading exhibited a high CH 3 OH yield of 4.3 mmol g cat. −1 h −1 with a selectivity of ~70% and a yield of 4.8 mmol g cat. −1 h −1 with an ultrahigh selectivity of ~80%, respectively (Fig. 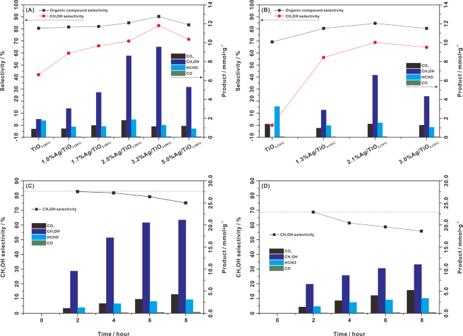Fig. 1: Photocatalytic CH4conversion with molecular O2. CH3OH selectivity and product yields for a series of Ag-loaded TiO2photocatalysts with predominantly exposedA{001} facets (0–5.0%Ag/TiO2 {001}) andB{101} facets (0–3.0%Ag/TiO2 {101}) under 2 h of irradiation. Time course for CH3OH selectivity and product yields forC3.2%Ag/TiO2 {001}andD2.1%Ag/TiO2 {101}under irradiation. Reaction conditions: 10 mg Ag/TiO2, 100 mL water, 2 MPa CH4, 0.1 MPa O2, 25 °C, light source: 300 W Xe lamp, light intensity of 450 mW/cm2. 1A and Table 1 ). For TiO 2 {101} , the 2.1%Ag loading shows an optimal CH 3 OH yield of 3.3 mmol g cat. −1 h −1 and a selectivity of ~68% (Fig. 1B and Table 1 ). Furthermore, with increasing irradiation time, the amounts of the total products (including CH 3 OH, HCHO, CO, and CO 2 ) increase gradually with relatively stable CH 3 OH selectivity (74–80%) in CH 4 photooxidation of 3.2%Ag/TiO 2 {001} . (Fig. 1C and Table 1 ). Similar results can also be found for 2.5%Ag/TiO 2 {001} (Supplementary Fig. S2 ). The optimal CH 3 OH yield and selectivity on 3.2%Ag/TiO 2 {001} are much superior to those of most reported photocatalytic systems for CH 4 oxidation to CH 3 OH (Supplementary Table S1 ). And we believe that this is the first study to achieve a high CH 3 OH yield and selectivity for CH 4 photooxidation with O 2 at room temperature. For 2.1%Ag/TiO 2 {101} , although the amount of the deep oxidation product (HCHO, CO, and CO 2 ) still increases with increasing irradiation time, the amount of CH 3 OH barely increases after 2 h of irradiation, which results in a significant decrease in CH 3 OH selectivity from 68% to 53% (Fig. 1D and Table 1 ). Therefore, it can be indicated that the mechanism for CH 4 photooxidation by O 2 on the {001} facet should be different from that on the {101} facet. The synergy between the cocatalyst Ag and the {001} facet can achieve selective and stable photocatalytic oxidation of CH 4 into CH 3 OH by O 2 . Table 1 Photocatalytic activity. Full size table Characterization of Ag/TiO 2 nanocatalysts To further clarify the correlation between photocatalytic performance and the crystal facet on Ag/TiO 2 nanocatalysts, high-resolution transmission electron microscopy (HRTEM, 3100FEF spectrometer) and X-ray photoelectron spectroscopy (XPS) were performed to validate the morphology and elemental structure of 2.5%Ag/TiO 2 {001} and 2.1% Ag/TiO 2 {101} . According to the HRTEM results, TiO 2 {001} exhibits a uniform square morphology with an average length of 54 nm and thickness of 4.6 nm (Fig. 2A ), and TiO 2 {101} possesses an octahedral morphology with an average size of 17 nm (Fig. 2D ). The lattice spacing parallel to the lateral facets and the top is 3.56 and 2.38 Å, corresponding to the {101} and {001} facets of anatase TiO 2 , respectively (Fig. 2B–E ). As such, it can be found that both TiO 2 {001} and TiO 2 {101} nanoparticles coexpose {001} and {101} facets, and the percentage of dominant facets should be ~87% of the {001} facet in TiO 2 {001} , and ~92% of the {101} facet in TiO 2 {101} . Furthermore, HRTEM clearly shows that the Ag cocatalyst with a particle size of ~1.5 nm was selectively photodeposited onto the {101} facet of 2.5%Ag/TiO 2 {001} as shown in Fig. 2A, B . The chemical states for the Ag species on 2.5%Ag/TiO 2 {001} were characterized by XPS (Fig. 2F ), and the Ag 3 d 5/2 peak observed at 368.0 eV can be associated with metal Ag nanoparticles. Similarly, on 2.1% Ag/TiO 2 {101} , the Ag cocatalyst was also selectively photodeposited onto the {101} facet. However, due to the larger {101} facet, Ag can be dispersed better and smaller (<1.0 nm) than that on 2.5%Ag/TiO 2 {001} (Fig. 2D, E ), which is reflected redshift observed for the Ag 3 d 5/2 peak (0.2 eV) in the XPS spectrum, as shown in Fig. 2F . According to the XPS results in Supplementary Fig. S3 , titanium atoms exist in the form of Ti 4+ –O bonds in both TiO 2 {101} and TiO 2 {001} [29] , as confirmed by the Ti 2 p 3/2 and 2 p 1/2 XPS peaks at 458.8 and 464.5 eV, and the O 1 s XPS spectra show two peaks at 530.0 and 531.4 eV ascribed to lattice oxygen in Ti–O 2 − –Ti bonds and OH groups on the surface of TiO 2 [30] . In addition, no fluorine or chlorine atoms are present on Ag/TiO 2 catalysts. The elemental composition of Ag and Ti was studied by energy dispersive spectroscopy (EDS), as shown in Supplementary Fig. S4 . In addition, according to N 2 adsorption and desorption experiments (Supplementary Fig. S5 ), the BET surface area of TiO 2 {101} (100.6 m 2 /g) is slightly higher than that of TiO 2 {001} (84.5 m 2 g −1 ). Due to the particle accumulation, both TiO 2 {101} and TiO 2 {001} are porous with similar pore diameters 14.3 and 14.9 nm, respectively. As such, compared with TiO 2 {101} , the higher photocatalytic activity and selectivity on TiO 2 {001} can be mainly ascribed to crystal plane and elemental structure rather than surface area and porosity. Fig. 2: Photocatalyst characterization. A – C HRTEM images of 2.5%Ag/TiO 2 {001} . D , E HRTEM images of 2.1%Ag/TiO 2 {101} . F Ag 3 d XPS spectra for 2.5%Ag/TiO 2 {001} (red line) and 2.1%Ag/TiO 2 {101} (black line). Full size image Reactive intermediate by operando and in situ characterization To gain insight into the different photocatalytic mechanisms for CH 4 photooxidation on the {001} and {101} facets of TiO 2 , reactive intermediates were detected by operando ATR-FTIR experiments on 2.5%Ag/TiO 2 {001} and 2.1% Ag/TiO 2 {101} in the aqueous phase. The change in the difference spectra before light irradiation was also taken as the reference and indicator. It is certain at first that all the spectra observed under different conditions showed no change before light irradiation (Supplementary Figs. S6 – S9 ). For the 2.5%Ag/TiO 2 {001} photocatalyst in the aqueous-phase saturated with Ar and O 2 (Ar + O 2 ) (Fig. 3A in 1st column), light irradiation led to the appearance of several peaks located at 943, 842, and 812 cm − 1 . The peaks in the 800–1000 cm − 1 region were specifically assigned in previous reports [31] , [32] to the O–O stretching of a surface peroxo species Ti–(OO) at 943 cm −1 [32] , [33] , Ti–OOH at 842 cm −1 [31] , and Ti–OO–Ti at 812 cm − 1 [32] , [34] , [35] , [36] . To validate this assignment, operando FTIR experiments were performed for the adsorption of H 2 O 2 on the surface of TiO 2 {001} over time, and it was confirmed that the signal in the region of 800–1000 cm − 1 corresponds to free and adsorbed H 2 O 2 (Supplementary Fig. S10 ). The intensities of the peaks at 943 and 812 cm − 1 increase immediately with the light irradiation time and drop down quickly after the light is turned off, suggesting that the intermediate species of Ti–(OO) and Ti–OO–Ti are photoinduced and metastable. Besides, these intermediate species show few changes with time under the light. However, when CH 4 was introduced into the aqueous-phase system instead of Ar (CH 4 + O 2 ), both peaks at 943 and 812 cm − 1 decreased significantly with light irradiation (Fig. 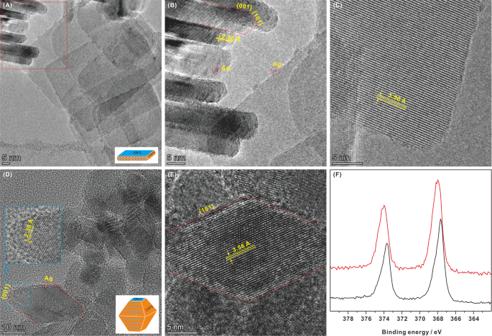Fig. 2: Photocatalyst characterization. A–CHRTEM images of 2.5%Ag/TiO2 {001}.D,EHRTEM images of 2.1%Ag/TiO2 {101}.FAg 3dXPS spectra for 2.5%Ag/TiO2 {001}(red line) and 2.1%Ag/TiO2 {101}(black line). 3A in 2nd column), suggesting the consumption of intermediate species (Ti–(OO) and Ti–OO–Ti) in the presence of CH 4 . Instead, two new peaks appear in the region of 1000–1100 cm − 1 , which can be assigned to the C–O stretching modes of CH 3 OH and Ti–O–CH 3 [37] . Fig. 3: Reactive intermediates on the {001} and {101} facets. A Operando ATR-FTIR matrix for 2.5%Ag/TiO 2 {001} and 2.1% Ag/TiO 2 {101} with a 4 mL aqueous phase in a (Ar + O 2 ) and (CH 4 + O 2 ) atmospheres before, during, and after light irradiation. B In situ ESR spectra for 2.5%Ag/TiO 2 {001} (left) and 2.1% Ag/TiO 2 {101} (right) with 300 µmol H 2 O loading in O 2 (bottom) and (CH 4 + O 2 ) (upper) atmospheres before and during light irradiation. We fit the ESR data with the easyspin programs. C Ex situ 17 O NMR spectra for 2.5%Ag/TiO 2 {001} (upper) and 2.1% Ag/TiO 2 {101} (lower) in a (CH 4 + 17 O 2 ) atmosphere before and after light irradiation. The signals marked by asterisks are spinning sidebands. We fit the 17 O NMR data with the Dimfit programs. Full size image Compared with the 2.5%Ag/TiO 2 {001} photocatalyst, no peak appears in the 800–1000 cm − 1 region for the 2.1%Ag/TiO 2 {101} photocatalyst in the aqueous phase with Ar + O 2 during light irradiation (Fig. 3A in 3rd column). It is suggested that the intermediates of Ti–(OO) and Ti–OO–Ti are not photoinduced on 2.1%Ag/TiO 2 {101} . A similar change in spectral behavior is observed for 2.1%Ag/TiO 2 {101} in the aqueous phase with CH 4 + O 2 during light irradiation (Fig. 3A in 4th column), except for the presence of the peaks in the region of 1000–1100 cm − 1 due to CH 3 OH and Ti–O–CH 3 formation during light irradiation. Notably, the peaks in the region of 1000–1100 cm − 1 on 2.1%Ag/TiO 2 {101} are much weaker than those on 2.5%Ag/TiO 2 {001} (Fig. 3A in 2nd and 4th columns) indicating that CH 4 activation on the {001} facet should make it easier to form CH 3 OH and Ti–OCH 3 . In addition, a new peak located at 966 cm − 1 can be assigned to the O–O stretching mode of CH 3 OOH (Fig. 3A in 4th column) [38] . We used in situ ESR spectroscopy to follow the formation of paramagnetic intermediates on the {001} and {101} facets (Fig. 3B ). For 2.5%Ag/TiO 2 {001} with 300 µmol H 2 O loading in a 24 µmol O 2 atmosphere, two sets of ESR signals appeared upon light irradiation (Fig. 3B , left). The strong signal at g = 1.9996 is associated with oxygen vacancies arising from trapped photoinduced holes at surface oxygen. According to previous reports [39] , [40] , the signal for orthorhombic symmetry at g zz = 2.023, g yy = 2.007, and g xx = 2.000 is ascribed to surface superoxide (Ti–O 2 • ) sites. O 2 • − is usually stabilized on a metallic cationic site so that the electrostatic interaction splits the 2π* antibonding orbitals by a certain amount (δ) due to the local cationic crystal field. The g zz value can be measured by the equation g zz = g e + 2 λ / δ , where λ is the spin–orbit coupling constant of oxygen [40] . As such, g zz = 2.023 indicates that O 2 • − is stabilized at the Ti sites for the oxygen vacancies. Combined with the operando FTIR results, the surface superoxide can be converted into surface peroxo species by the reduction of photoinduced electrons. However, when 30 µmol CH 4 was introduced into the O 2 –Ag/TiO 2 {001} system ((CH 4 + O 2 )–Ag/TiO 2 {001} ), both ESR signals decreased obviously upon light irradiation, indicating the consumption of paramagnetic intermediates (oxygen vacancies and Ti–O 2 • ) in the presence of CH 4 . Compared with 2.5%Ag/TiO 2 {001} , no surface superoxide appears for 2.1%Ag/TiO 2 {101} with a 300 µmol H 2 O loading in a 24 µmol O 2 atmosphere during light irradiation (Fig. 3B , right), except for a small number of oxygen vacancies associated with the signal at g = 1.9996. Furthermore, the amount of oxygen vacancies does not change in the presence of 30 µmol CH 4 , indicating that oxygen vacancies are not involved in CH 4 photooxidation by O 2 on 2.1%Ag/TiO 2 {101}. In addition, the pair of signals at g = 2.03 and 1.96 should be assigned to the background signal of in situ ESR tube (Supplementary Fig. S11 ). Ex-situ 17 O MAS NMR experiments were used to follow the transfer and evolution of oxygen in CH 4 photooxidation by 17 O 2 on TiO 2 photocatalysts (Fig. 3C ). For 2.5%Ag/TiO 2 {001} in a 24 µmol 17 O 2 and 30 µmol CH 4 atmosphere, three NMR signals appeared after 0.5 h of light irradiation. According to the previous reports [41] , the resonances at 480–570 ppm should arise from three coordinated oxygen species in the bulk of TiO 2 ; the peaks at higher frequencies (600–750 ppm) can be assigned to two coordinated oxygen species on the surface of TiO 2 ; the signals at much lower frequencies (100–300 ppm) can be attributed to hydroxyl groups (Ti–OH); the signals at −100–10 ppm can be attributed to adsorbed H 2 O. As such, the signals observed at −24 and 180 ppm are associated with H 2 17 O and surface terminal hydroxyl (Ti– 17 OH), respectively (Fig. 3C , upper). Due to the deshielding effect of CH 3 , the 17 O NMR signal of Ti–OCH 3 should shift to a lower field than that of Ti–OH. Accordingly, we assign the 17 O NMR signal at 263 ppm to Ti–OCH 3 (Fig. 3C , upper), which is in good agreement with the formation of –OCH 3 in the operando IR experiment for CH 4 oxidation. Similar results are obtained on 2.1%Ag/TiO 2 {101} in a 24 µmol 17 O 2 and 30 µmol CH 4 atmosphere before and after light irradiation (Fig. 3C , lower). However, the 17 O signals at 180 ppm and 263 ppm are much lower than those for 2.5%Ag/TiO 2 {001} , indicating that the O transfer efficiency from O 2 to Ti–OCH 3 and Ti–OH on the {001} facet in the photoreaction is much higher than that on the {101} facet. Combined with the operando FTIR and in situ ESR results, this can be attributed to the difference in the photocatalytic mechanism between the {001} and {101} facets, rather than the difference in the catalytic activity, because of the difference in reactivity (Fig. 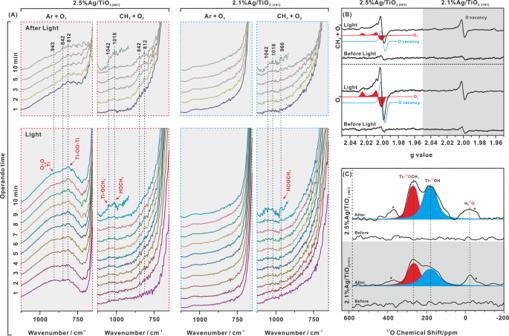Fig. 3: Reactive intermediates on the {001} and {101} facets. AOperando ATR-FTIR matrix for 2.5%Ag/TiO2 {001}and 2.1% Ag/TiO2 {101}with a 4 mL aqueous phase in a (Ar + O2) and (CH4+ O2) atmospheres before, during, and after light irradiation.BIn situ ESR spectra for 2.5%Ag/TiO2 {001}(left) and 2.1% Ag/TiO2 {101}(right) with 300 µmol H2O loading in O2(bottom) and (CH4+ O2) (upper) atmospheres before and during light irradiation. We fit the ESR data with the easyspin programs.CEx situ17O NMR spectra for 2.5%Ag/TiO2 {001}(upper) and 2.1% Ag/TiO2 {101}(lower) in a (CH4+17O2) atmosphere before and after light irradiation. The signals marked by asterisks are spinning sidebands. We fit the17O NMR data with the Dimfit programs. 1 ) is far from matching the difference in the O transfer efficiency. 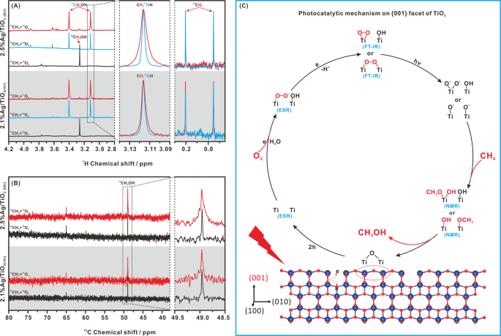Fig. 4: Photocatalytic mechanism. A1H andB13C NMR spectra for the product obtained from photocatalytic CH4oxidation at a 4 h reaction time using 50 mL water, 80 kPa CH4, 20 kPa O2, and 10 mg Ag/TiO2.CProposed photocatalytic mechanism for CH4oxidation by O2on the {001} facets of TiO2. Distinct photocatalytic mechanism of CH 4 oxidation by O 2 on the {001} facet To detect the direct participation of CH 4 and O 2 in the formation of CH 3 OH, isotope labeling NMR experiments using 13 CH 4 and 17 O 2 were conducted under 80 kPa 13 CH 4 mixed with 20 kPa 17 O 2 on 2.5%Ag/TiO 2 {001} and 2.1% Ag/TiO 2 {101} in 50 mL water for 4 h. Figure 4A shows the 1 H NMR spectra for the product obtained from photocatalytic CH 4 oxidation in various atmospheres. For 2.5%Ag/TiO 2 {001} in a 12 CH 4 and 16 O 2 atmosphere, the strong peak at 3.26 ppm corresponds to 12 CH 3 OH, and the weak peak at 3.77 ppm corresponds to trace 12 CH 3 OOH. Using 13 CH 4 instead of 12 CH 4 , both peaks split into two peaks due to 1 H– 13 C J coupling (~140 Hz) for the methyl groups in the formed 13 CH 3 OH (3.40 and 3.12 ppm) and 13 CH 3 OOH (3.62 and 3.91 ppm) (Fig. 4A , upper). Similar results are also obtained on 2.1%Ag/TiO 2 {101} (Fig. 4A , lower). It can be indicated that the product CH 3 OH indeed originates from CH 4 conversion on both 2.5%Ag/TiO 2 {001} and 2.1% Ag/TiO 2 {101} . Interestingly, when the reaction was carried out on 2.5%Ag/TiO 2 {001} in a 13 CH 4 and 17 O 2 atmosphere, the FWHM (full width at half maximum) for the 13 CH 3 OH signal obviously increased (Fig. 4A , upper). It should be noted that the FWHM of the signal for dissolved 13 CH 4 (0.20 and −0.04 ppm) in the 13 CH 4 and 17 O 2 atmosphere is consistent with that of dissolved 13 CH 4 in the 13 CH 4 and 16 O 2 atmosphere (Fig. 4A , upper). Thus, the widening of the 13 CH 3 OH signal is due to weak J coupling (1.96 Hz) between the methyl proton and 17 O, rather than any error related to the spectrometer and operation. On the other hand, when the reaction was carried out on 2.1% Ag/TiO 2 {101} in a 13 CH 4 and 17 O 2 atmosphere, the FWHM for the signal for the product 13 CH 3 OH barely increased compared with that of the product 13 CH 3 OH in a 13 CH 4 and 16 O 2 atmosphere (Fig. 4A , lower). Similar results were also found from the 13 C NMR spectra (Fig. 4B ). For Ag/TiO 2 in the 13 CH 4 and 16 O 2 atmosphere, the two 13 C NMR signals at 48.97 and 65.03 ppm can be attributed to 13 CH 3 OH and 13 CH 3 OOH, respectively, which further proves that the product CH 3 OH indeed originated from CH 4 conversion on both 2.5%Ag/TiO 2 {001} and 2.1% Ag/TiO 2 {101} . When the reaction was carried out on Ag/TiO 2 in a 13 CH 4 and 17 O 2 atmosphere, the obvious peak broadening, originating from 13 C– 17 O J coupling only occurred for the signal for 13 CH 3 OH generated by 2.5%Ag/TiO 2 {001} (Fig. 4B , upper) but was barely observed for the signal for 13 CH 3 OH generated by 2.1% Ag/TiO 2 {101} (Fig. 4B , lower). Combined with the results from 1 H NMR experiments, it can be indicated that the oxygen in the CH 3 OH product mainly originates from the O 2 in the photocatalytic CH 4 oxidation on the {001} facet, while the oxygen in the CH 3 OH product should mainly originate from H 2 O and the surface oxygen of TiO 2 in the photocatalytic CH 4 oxidation on the {101} facet. Fig. 4: Photocatalytic mechanism. A 1 H and B 13 C NMR spectra for the product obtained from photocatalytic CH 4 oxidation at a 4 h reaction time using 50 mL water, 80 kPa CH 4 , 20 kPa O 2 , and 10 mg Ag/TiO 2 . C Proposed photocatalytic mechanism for CH 4 oxidation by O 2 on the {001} facets of TiO 2 . Full size image As in the previous reports [2] , [7] , [9] , [42] , the primary step of CH 4 activation on typical oxide semiconductors should involve a reaction with surface O − radical ions. When a TiO 2 {101} sample is illuminated under UV irradiation, the surface oxygen (Ti–O–Ti) captures one photoinduced hole to form Ti–O • [2] , [3] , [4] . As O − is present on typical TiO 2 and ZnO [2] , [9] , Ti–O • can easily react with CH 4 and H 2 O to form •CH 3 and •OH: 
    Ti-O^∙+CH_4→Ti-OH+∙CH_3,
 (1) 
    Ti-O^∙+^-OH→Ti-OH+∙OH,
 (2) which was proven by ESR for 2.1% Ag/TiO 2 {101} in an aqueous solution (Supplementary Fig. S12 ). The active •CH 3 can couple with the surface O − and •OH to form Ti–OCH 3 and CH 3 OH, as evidenced in the IR range of 1000–1100 cm − 1 (Fig. 3A in 4th column). This is the reason why the oxygen in the CH 3 OH product mainly originates from H 2 O and Ti–O–Ti rather than O 2 in the photocatalytic CH 4 oxidation on 2.1% Ag/TiO 2 {101} (Fig. 4A, B ). The O 2 can be reduced by photoinduced electrons to form superoxide anion radicals (O 2 • − ), which can easily react with •CH 3 to form CH 3 OOH associated with the IR signal at 966 cm − 1 (Fig. 3A in 4th column) [2] , [9] , [42] : 
    O_2+e→O_2^∙ -,
 (3) 
    ∙CH_3+O_2^∙ -+H^+→CH_3OOH∙
 (4) CH 3 OOH can readily decompose into formaldehyde (HCHO) and H 2 O [2] , [9] , and HCHO and CH 3 OH can be overoxidized to CO 2 and H 2 O by •OH radicals. Thus, as long as •CH 3 and •OH radicals occur in photocatalytic CH 4 oxidation, overoxidation should be unavoidable. It has been found that the Ti–O–Ti bond angles of the {001} facets are more distorted than those of the {101} facets [21] , and there are much more pentacoordinated Ti 4+ sites present on the {001} facets than that on the {101} facet [21] , [24] . All this leads to a higher surface energy (0.90 J m −2 ) on {001} facets than that (0.44 J m −2 ) on {101} facets [23] . In order to further prove the difference of the activity of oxygen sites and the formation of intermediates (oxygen (O) vacancy and surface peroxide species) on {001} and {101} facet of TiO 2 , the theoretical calculation has been performed (Supplementary Fig. S13 ). The energy ( E f ) required for the formation of O vacancy on {001} facet is much lower than that on the {101} facet, and the energy ( E ads ) released by O 2 adsorption on O vacancy of {001} facet is much higher than that on O vacancy of {101} facet. In one word, the energy (2.717 eV) required for the formation of peroxide intermediate by O 2 adsorption on {001} facet is much lower than that (3.983 eV) on {101} facet. Therefore, it can be concluded that, firstly, the O centers of the {001} facet are more active than those of the {101} facet, which is favorable for the formation of O vacancies on the {001} facet upon light irradiation, as confirmed by the ESR signal at g = 1.9996 in Fig. 3B ; secondly, it should be easier to form peroxide intermediates by O 2 adsorption on {001} facet, as confirmed by the operando FTIR experiment in Fig. 3A . Thus, unlike CH 4 activation on the {101} facet, the primary step of CH 4 activation on the {001} facet should be the oxidation of surface oxygen by photoinduced holes to form oxygen vacancies: 
    Ti-O-Ti + 2 h → Ti Ti,
 (5) which results in a distinct catalytic mechanism appearing on the {001} facet (Fig. 4C ). The oxygen vacancy can stabilize the superoxide radical (O 2 • − ), which should be formed by O 2 reduction by photoinduced electrons, as in reaction 3, to form surface superoxide (Ti–O 2 • ): 
    Ti Ti+O_2^∙ -→Ti-OO^∙ Ti
 (6) which is associated with the ESR signals at g zz = 2.023, g yy = 2.007, and g xx = 2.000 (Fig. 3B ). The surface superoxide can capture photoinduced electrons to form two types of surface peroxides (Ti–OO–Ti and Ti–(OO)): 
    Ti-OO^∙ Ti +e → Ti-OO-Ti,
 (7) which corresponds to the appearance of O–O stretching bands at 812 and 943 cm − 1 that show increased intensity with light irradiation time in the operando FTIR experiment, respectively (Fig. 3A in 1st column). With the presence of CH 4 , both Ti–OO–Ti and Ti–(OO) decrease significantly upon light irradiation (Fig. 3A in 2nd column). Theoretically, the dissociation barrier for the surface peroxides into Ti–O • pairs on the {001} facet of anatase TiO 2 is 1.0–1.4 eV, which can be overcome by the photon energy available from UV and visible light irradiation [43] : 
    Ti-OO-Ti +hν→Ti-O^∙ ^∙O-Ti. (8) The Ti–O • pairs can split CH 4 to generate adjacent surface methoxyl and hydroxyl groups (Ti–OCH 3 HO–Ti), which are associated with the NMR signals observed 263 and 180 ppm, respectively (Fig. 3C ), subsequently releasing CH 3 OH: 
    Ti-O^∙ ^∙O-Ti+CH_4→Ti-OCH_3HO-Ti→Ti-O-Ti+CH_3OH. (9) This should be the reason why the oxygen in the CH 3 OH product mainly originates from O 2 rather than H 2 O and Ti–O–Ti on 2.5% Ag/TiO 2 {001} (Fig. 4 A, B ), with almost no •CH 3 and •OH generated in the photocatalytic CH 4 oxidation on 2.5% Ag/TiO 2 {001} (Supplementary Fig. S12 ). Obviously, this reaction path can effectively hinder the formation of CH 3 OOH. According to the ESR spectra (Supplementary Fig. S12 ), there are no •OH species present in the photocatalytic CH 4 oxidation on 2.5% Ag/TiO 2 {001} , which can greatly reduce the overoxidation of CH 3 OH by •OH [2] . In addition, the presence of water in the reactions could promote the desorption of methoxyl/methanol from the surface of catalysts into an aqueous solution to avoid overoxidation of methanol to CO and CO 2 [15] , [16] , [17] , since the product CH 3 OH can physically or chemically adsorb onto the photocatalyst surface [4] , and can be further oxidized with the surface-active species (such as Ti–O • , peroxides, and superoxide) to form CO and CO 2 [9] , [10] . Thus, the aqueous phase is important to improve CH 3 OH selectivity in a photocatalytic CH 4 oxidation reaction. The proposed mechanism can further shed light on the results obtained for the photocatalytic activity and selectivity relative to the Ag loading amount on both TiO 2 {001} and TiO 2 {101} . As observed in Fig. 1 A, B , the initial increase in Ag loading can increase the photocatalytic activity and selectivity for both TiO 2 {001} and TiO 2 {101} . To get insight into the role of Ag, the operando ATR-FTIR experiments on TiO 2 {001} and TiO 2 {101} have been performed (Supplementary Fig. S14 ). Similar to 2.5%Ag/ TiO 2 {001} , light irradiation also led to two types of surface peroxo intermediates (Ti–OO–Ti and Ti–(OO)) for the TiO 2 {001} in the aqueous phase saturated with Ar and O 2 (Ar + O 2 ). On the other hand, similar to 2.1%Ag/TiO 2 {101} , almost no peak appears in the 800–1000 cm − 1 region for the TiO 2 {101} in the aqueous phase with Ar + O 2 during light irradiation. It can be indicated that the formation of surface peroxo intermediates mainly occurred on the {001} facet of TiO 2 . The in situ ESR experiments were used to follow the formation of paramagnetic intermediates on TiO 2 {001} and TiO 2 {101} (Supplementary Fig. S15 ). Different from 2.5%Ag/ TiO 2 {001} , no surface superoxide (Ti–O 2 • ) was observed on both TiO 2 {001} and TiO 2 {101} in the presence of 300 μmol H 2 O and 24 μmol O 2 during light irradiation, while a small number of oxygen vacancies was formed on TiO 2 {001} . It can be indicated that Ag loading contributes to the formation of Ti–O 2 • on TiO 2 {001} . This may have two reasons: firstly, Ag as a cocatalyst can trap the photogenerated electrons to reduce molecular O 2 to form O 2 − species; secondly, the electron trapping on cocatalyst Ag can effectively improve the separation of photogenerated electrons and holes, which can lead to the increase of O vacancy formation arisen from the oxidation of surface oxygen by photogenerated hole on the {001} facet of TiO 2 (Fig. 3B ). As a result, the observable O 2 − species is stabilized at the O vacancy on the {001} facet of TiO 2 loaded with Ag (Fig. 3B ). In addition to the role of Ag in separating the electron-hole pairs to increase the activity, more Ag loading can reduce the exposed area of the {101} facet since the Ag is mainly photodeposited on the {101} facet. Instead, the {001} facet will continue to be exposed to the solution, resulting in superior selectivity. However, excessive loading of Ag will decrease the activity because of the intrinsic light absorption by Ag, while the selectivity can remain high since the {001} facet can still be exposed to the solution. In summary, we report the photocatalytic oxidation of CH 4 into CH 3 OH by molecular O 2 on anatase TiO 2 . To compare the microstructure and catalytic mechanism on the {001} and {101} facets of TiO 2 , two types of TiO 2 with predominantly exposed {001} or {101} facets were prepared. By selectively photodepositing a Ag cocatalyst onto the {101} facet of TiO 2 to facilitate the separation and transfer of photoinduced carriers, the CH 3 OH yield can be promoted significantly. According to studies based on operando FTIR, in situ ESR, and NMR techniques, completely different catalytic mechanisms exist for CH 4 photooxidation by O 2 on the {001} and {101} facets. It was found that oxygen vacancies on {001} facets are generated in a straightforward manner by photoinduced holes and that these photogenerated oxygen vacancies can stabilize superoxide radicals (Ti–O 2 • ). Ti–O 2 • can capture photoinduced electrons to form surface peroxides (Ti–OO–Ti and Ti–(OO)), and the surface peroxides dissociate into Ti–O • pairs, which can split CH 4 to release CH 3 OH directly. This distinct catalytic mechanism effectively avoids the formation of •CH 3 and •OH, which are the main factors leading to overoxidation and are generally formed on the {101} facet. Thus, the optimized {001} facet-dominated TiO 2 sample shows an impressively high CH 3 OH yield of 4.8 mmol g −1 h −1 with high CH 3 OH selectivity of ~80%. This study will provide a strategy to avoid overoxidation in CH 4 reforming to CH 3 OH in other photocatalysts by controlling the generation of photoinduced oxygen vacancies. Sample preparation The anatase TiO 2 with predominantly exposed {001} facets (TiO 2 {001} ) were prepared according to the previous report [44] . 25 mL of Ti(OBu) 4 and 4 mL of hydrofluoric acid solution were mixed in a dried Teflon autoclave with a capacity of 100 mL, and then kept at 180 °C for 24 h. After being cooled to room temperature, the white powder was separated by high-speed centrifugation and washed with ethanol, 0.1 M NaOH aqueous solution, and deionized water several times to remove F − on the surface. The anatase TiO 2 with predominantly exposed {101} facets (TiO 2 {101} ) were prepared according to the previous report [45] . Firstly, for the preparation of Ti(OH) 4 precursor, 6.6 mL of TiCl 4 was added to aqueous HCl (0.4 mol L −1 ) drop by drop under strong stirring in an ice bath to obtain an aqueous TiCl 4 . This TiCl 4 aqueous was then added to aqueous NH 3 ·H 2 O (5.5 wt.%) drop by drop under stirring. White Ti(OH) 4 precipitate could be formed during the process. Afterward, the aqueous NH 3 ·H 2 O (4.0 wt.%) was added to adjust the pH value to 6–7. After aging at room temperature for 2 h, the suspension was centrifuged, and the precipitate was washed with ethanol, 0.1 M NaOH aqueous solution, and deionized water several times to remove Cl − on the surface. 4.0 g the fresh Ti(OH) 4 precursor was first dispersed in the mixture of 30 mL deionized water and 30 ml isopropanol. After stirring and ultrasonic treatment, the suspension was transferred to a 100 mL Teflon-lined autoclave and heated for 24 h at 180 °C. The products were collected by centrifugation and washed with deionized ethanol one time and water three times. According to the EDX of TiO 2 {101} and TiO 2 {001} (Supplementary Fig. S16 ), there is no fluorine or chlorine atoms present on these TiO 2 . The Ag-loaded TiO 2 catalyst was prepared by in situ photodeposited reactions of AgNO 3 with TiO 2 . Briefly, 0.4 g of the prepared TiO 2 was suspended in an anaerobic aqueous solution containing deionized water (20.0 mL), CH 3 OH (5.0 mL), and a certain number of AgNO 3 . After 0.5 h irradiation under 300 W Xe lamp, the products were collected via centrifugation, then washed by water and dried at 60 °C. Characterization A homemade spectral cell for attenuated total reflectance (ATR) Fourier transform infrared spectroscopy (FTIR) experiments is shown in Supplementary Fig. S17 [32] . An internal reflection element (IRE) made of ZnSe (size: 50 mm × 20 mm × 3 mm, incident angle: 60°) was obtained from Pier Optics Co., Ltd. Japan. 20 mL TiO 2 suspensions of 5 mg mL − 1 in ethanol were drop casted on the IRE surface and dried in air. The IRE with TiO 2 coating was then set into the homemade spectral cell. 4 mL of water was purged by the gas for different purposes and was then injected into the cell. Before the Operando ATR-FTIR experiments, the cell was kept in dark for 5 min. An FTIR spectrometer (FT/IR-6300, Jasco Inc.) with liquid nitrogen cooled MCT detector was used and purged by dry nitrogen before ATR-FTIR experiments. The absorbance spectra ranged from 4000 to 500 cm − 1 were obtained by repeated 32 scans with a resolution of 4 cm − 1 and a processing time of 30 s. The background was monitored and recorded in every minute of 5 min before the light illumination. Thereafter, the spectra were obtained at every minute of 10 min with light illumination and after light illumination. 17 O solid-state NMR spectra were acquired at 18.8 T on the Bruker Avance III spectrometers, equipped with a 4 mm double-resonance probe. The Larmor resonance frequencies for the 1 H and 17 O resonances were 800.4 and 108.5 MHz, respectively. 17 O MAS NMR spectra were acquired using a typical π/2 pulse length of 2.5 μs, with a recycle delay of 1.0 s and a 1 H decoupling field strength of 130 kHz. The experiments were carried out with a MAS frequency of 13.5 kHz. 120,000 scans were accumulated to acquire each spectrum. The chemical shifts of 17 O resonance signals were referred to as liquid H 2 17 O. Prior to ex-situ 17 O NMR measurements, CH 4 (30 μmol) and 17 O 2 (20μmol) were introduced into a glass ampule containing 0.05 g TiO 2 catalyst under vacuum at the liquid N 2 temperature, and then the glass ampule was sealed off. The photoreaction was performed in the sealed ampule under successive irradiation by a 300 W Xe lamp, and then the ampule was transferred into the rotor for the ex situ NMR measurements. A homemade spectral cell for in situ electron spin resonance (ESR) experiments is shown in Supplementary Fig. S18 . In situ ESR experiments were carried at X-band using a JOEL FA 2000 spectrometer. The microwave frequency was 9.1 GHz, the modulation amplitude was 0.1 mT, the microwave power was 5 mW and the experimental temperature was 25 °C. The g values of the radical species were referenced to Mn-marker. The Mn-marker is Mn 2+ in the CaO with g = 2.0009. Photocatalytic measurements The photocatalytic methane oxidation reaction tests were conducted in a 230 mL batch reactor equipped with a quartz window to allow light irradiation. 10 mg catalyst was dispersed in 100 mL water by ultrasonication for 10 min. Then, the mixture was added into a glass cell with a volume of 30 mL, and the glass cell was placed in the batch reactor. The actual working volume decreased to 100 mL. The batch reactor was purged with O 2 (purity, 99.99995%) for 15 min to exhaust air. After that, the reactor vessel was pressurized with 0.1 MPa O 2 and 2 MPa CH 4 (purity, 99.9995%). Subsequently, the reactor was loaded into a cold-water bath, and the solution was stirred at 1200 rpm. 300 W Xe lamp was used as the light source with wavelength ranging from 300 to 500 nm and the light intensity of 450 mW cm −2 . A thermocouple was inserted into the solution to directly detect the temperature of the liquid solution. During the reaction process, the temperature of the liquid solution was maintained at 25 °C. After the reaction, the reactor was cooled in an ice bath to a temperature below 10 °C. Then the gas product was collected, and the concentrations of gas products were analyzed by gas chromatograph (GC, Shimadzu) equipped with methanizer and flame ionization detector. The liquid phase of the reaction mixture product was collected by centrifugation. The liquid product was analyzed by nuclear magnetic resonance spectroscopy (NMR) and the colorimetric method.